Sublinear binocular integration preserves orientation selectivity in mouse visual cortex Inputs from the two eyes are first combined in simple cells in the primary visual cortex. Consequently, visual cortical neurons need to have the flexibility to encode visual features under both monocular and binocular situations. Here we show that binocular orientation selectivity of mouse simple cells is nearly identical to monocular orientation selectivity in both anaesthetized and awake conditions. In vivo whole-cell recordings reveal that the binocular integration of membrane potential responses is sublinear. The sublinear integration keeps binocularly evoked depolarizations below threshold at non-preferred orientations, thus preserving orientation selectivity. Computational simulations based on measured synaptic conductances indicate that inhibition promotes sublinear binocular integration, which are further confirmed by experiments using genetic and pharmacological manipulations. Our findings therefore reveal a cellular mechanism for how visual system can switch effortlessly between monocular and binocular conditions. The same mechanism may apply to other sensory systems that also integrate multiple channels of inputs. Diverse behavioural tasks require the brain to integrate signals from multiple input channels. Neurons in the sensory cortex, for example, receive inputs from bilateral sensory organs [1] , other sensory modalities [2] and motor areas [3] . Because the number of active input channels varies in real time, cortical neurons must have the flexibility to cope with various situations when different channels are recruited. In particular, cortical neurons that encode certain stimulus features through individual channels need to preserve their selectivity when more input channels are added. How this is achieved is a fundamental question in sensory neurobiology and its underlying cellular mechanism is largely unknown. In the visual system, the inputs from the two eyes are first combined in simple cells in the primary visual cortex (V1) (ref. 4 ). In addition to binocularity, another important functional property emerges in simple cells, namely, the orientation selectivity [5] . When stimulated monocularly, simple cells in adult V1 are tuned to similar orientations through the two eyes [6] , [7] , [8] . Their selectivity must be maintained when they are stimulated through both eyes, so that visual perception remains unchanged when switching between binocular and monocular conditions. The preservation of binocular orientation selectivity is not a trivial or automatic process. This is because although the spiking output of simple cells is highly selective, their synaptic inputs are less so. Each simple cell typically receives inputs across all orientations, with only a moderate bias towards its preferred orientation. Action potential threshold amplifies the suprathreshold responses to the preferred orientations and masks the subthreshold responses to other orientations [9] , [10] , [11] . In other words, the membrane potential depolarization at each orientation determines the degree of selectivity. Consequently, whether binocular orientation tuning can be preserved depends critically on how the synaptic inputs from the two eyes are integrated. Binocular integration in V1 has been studied in cats and primates for decades. However, these studies have mostly focused on either binocular disparity or binocular rivalry, instead of the preservation of orientation tuning. To study binocular disparity, visual stimuli are typically fixed at the preferred orientation of the recorded cell, while various interocular differences in the stimulus are introduced to test the cell’s selectivity [12] , [13] , [14] . For binocular rivalry, different patterns of stimuli are again used to stimulate the two eyes [15] . For example, in the paradigm of ‘interocular cross-orientation suppression’, the stimulus is fixed at the preferred orientation through one eye and various orientations are delivered to the other eye to probe their influence [16] . In neither case has binocular orientation tuning been quantitatively characterized, although it has long been shown that V1 binocular response is qualitatively selective [5] . Importantly, the cellular mechanism for preserving binocular orientation tuning has not been revealed. Mice have emerged as a useful model in vision research, due to the powerful genetic tools to manipulate neuronal circuits and development. Similar to higher mammals, mouse simple cells are highly selective [17] . Recent studies have begun to untangle synaptic mechanisms of monocular orientation selectivity in mice [10] , [11] , [18] , [19] , [20] . Binocular orientation tuning in mice, however, has never been examined. In this study, we have conducted extracellular and intracellular recordings in mouse V1 to investigate binocular integration in simple cells and its influence on orientation tuning. We first find that in both anaesthetized and awake mice, simple cells maintain their orientation tuning of spiking output in response to binocular stimulation. We then reveal that these cells integrate their membrane potential responses sublinearly, and the sublinear integration is critical for preserving the binocular orientation tuning. Furthermore, computational simulations and experimental data with genetic and pharmacological manipulations indicate a role of synaptic inhibition in promoting sublinear integration. Finally, we show that the inter-hemispherical interactions between the two visual cortices enhance responses to the ipsilateral eye, but do not affect binocular integration. Together, our results illustrate a cellular mechanism that preserves orientation tuning while integrating binocular inputs, which might be generalizable to other multi-channel sensory processes. Preserved binocular orientation selectivity in mouse V1 We first made extracellular single-unit recordings in the binocular zone of V1 in anaesthetized mice. For each cell, its binocular tuning was examined with both eyes exposed to sinusoidal gratings of varying drifting directions and spatial frequencies. Monocular tuning was also determined separately for each eye at the spatial frequency that elicited the maximal binocular response. We focused our study on the simple cells ( n =27/60), as they are the first stage of binocular integration in the cortex. The vast majority of these neurons were highly selective and tuned to similar orientations through the two eyes ( Fig. 1a and Supplementary Fig. S1 ), consistent with our previous report [8] . The strong orientation selectivity was preserved when responding to binocular stimulation (for example, Fig. 1a ), with the averaged monocular and binocular orientation tuning curves nearly identical ( Fig. 1b ). We also calculated an orientation selectivity index (OSI) and a modified circular variance (CV) to quantify individual tuning curves ( Supplementary Methods ). Both OSI ( Fig. 1c–e ) and CV ( Fig. 1f–h ) were similar between monocular and binocular responses across the population. 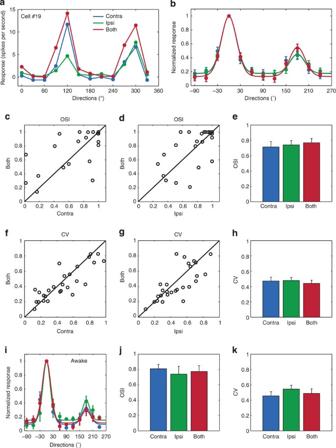Figure 1: Similar binocular and monocular orientation tuning in mouse V1 simple cells. (a) Monocular and binocular spiking responses at various directions of an example simple cell through the contralateral eye (‘Contra’, in blue), ipsilateral eye (‘Ipsi’, in green) and both eyes (red). The same colours are used to indicate different eye conditions in all figures unless otherwise stated. (b) Mean normalized monocular and binocular tuning curves (n=27). (c,d) Comparison between binocular and monocular OSI of individual cells. (e) Binocular and monocular OSIs. No significant difference was detected (0.71±0.07 for contralateral, 0.74±0.06 for ipsilateral and 0.77±0.06 for both eyes,n=27;P>0.2 for all comparisons, pairedt-test). (f–h) Monocular and binocular CV. No significant difference was detected (0.47±0.05 for contralateral, 0.48±0.04 for ipsilateral and 0.44±0.05 for both eyes,P>0.2, pairedt-test). (i–k) Normalized tuning curves, mean OSIs and mean CVs of cells recorded in awake mice. No significant difference between monocular and binocular orientation tuning, as in the anaesthetized condition (OSI=0.81±0.06 for contra, 0.74±0.10 for ipsi and 0.77±0.07 for both; CV=0.46±0.05 for contra, 0.54±0.05 for ipsi and 0.49±0.06 for both,P>0.5 for all comparisons,n=27, pairedt-test). Pooled data were presented as mean±s.e.m. Figure 1: Similar binocular and monocular orientation tuning in mouse V1 simple cells. ( a ) Monocular and binocular spiking responses at various directions of an example simple cell through the contralateral eye (‘Contra’, in blue), ipsilateral eye (‘Ipsi’, in green) and both eyes (red). The same colours are used to indicate different eye conditions in all figures unless otherwise stated. ( b ) Mean normalized monocular and binocular tuning curves ( n =27). ( c , d ) Comparison between binocular and monocular OSI of individual cells. ( e ) Binocular and monocular OSIs. No significant difference was detected (0.71±0.07 for contralateral, 0.74±0.06 for ipsilateral and 0.77±0.06 for both eyes, n =27; P >0.2 for all comparisons, paired t -test). ( f – h ) Monocular and binocular CV. No significant difference was detected (0.47±0.05 for contralateral, 0.48±0.04 for ipsilateral and 0.44±0.05 for both eyes, P >0.2, paired t -test). ( i – k ) Normalized tuning curves, mean OSIs and mean CVs of cells recorded in awake mice. No significant difference between monocular and binocular orientation tuning, as in the anaesthetized condition (OSI=0.81±0.06 for contra, 0.74±0.10 for ipsi and 0.77±0.07 for both; CV=0.46±0.05 for contra, 0.54±0.05 for ipsi and 0.49±0.06 for both, P >0.5 for all comparisons, n =27, paired t -test). Pooled data were presented as mean±s.e.m. Full size image Recent studies have shown that the animal’s wakefulness could influence V1 activity [21] , [22] . We thus compared binocular and monocular responses in the V1 of head-fixed awake mice. Just like in the anaesthetized condition, simple cells from the awake mice displayed similar monocular and binocular orientation tuning ( Fig. 1i–k ), confirming that V1 neurons maintain their orientation selectivity when viewing through both eyes. Sublinear binocular integration of spiking responses We also compared the responsiveness of simple cells between monocular and binocular conditions. In the anaesthetized animals, most binocular responses were smaller than the linear summation of the two monocular responses at the same stimulus conditions ( Fig. 2a ). Consequently, the integration ratio, defined as the binocular response over the sum of the two monocular ones, was significantly less than 1 over the entire range of response magnitude ( Fig. 2c ), indicating a sublinear binocular integration. The same integration ratio was observed for simple cells in layer 4, the cortical layer that receives direct eye-specific inputs from the dorsal lateral geniculate nucleus (dLGN) ( Supplementary Fig. S2 ), indicating that sublinear integration of binocular inputs takes place at the first stage of convergence and then propagates throughout the visual cortex. Furthermore, the integration ratio in awake mice was similar to the anaesthetized ones ( Fig. 2b ). Notably, in a substantial portion of cells (30%, n =8/27 in anaesthetized mice, and 42%, n =5/12 in awake mice), the binocular response at the preferred orientation was even weaker than the stronger monocular response, indicating an interocular suppression. These results thus demonstrate that the binocular integration of spiking responses in mouse V1 is sublinear and sometimes even suppressive. In other words, the responsiveness of visual cortical cells is restricted within a narrow range when more inputs are added. 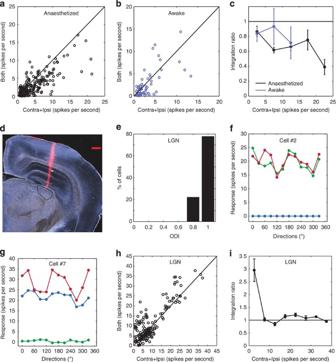Figure 2: Sublinear binocular integration of spiking responses. (a) Comparison of binocular spiking response and the linear summation of monocular responses in anaesthetized mice. Most points fell below the unity line, indicating a sublinear binocular integration. (b) Comparison of binocular spiking response and the linear summation of monocular responses in awake mice. (c) Binocular integration ratio in anaesthetized (black) and awake (blue) conditions. Integration ratio was plotted against the response magnitude, grouped at a bin width of 5 spikes per second. (d) A coronal section confirming recording site in the dLGN. The electrode track was marked with DiI (red). Four pictures were assembled to obtain the whole image. The dLGN was approximately marked with a black outline. Scale bar, 400 μm. (e) Distribution of ocular dominance index (ODI). Most cells had ODI of 1, indicating that they were monocular. (f–g) Two example dLGN cells in response to contralateral (blue), ipsilateral (green) and both eye stimulation (red). One cell was responsive to the contralateral eye (g), the other to the ipsilateral eye (f). The monocular response did not change much upon opening the other eye for most cells (f), but increased for some (g). Note that although dLGN cells were much less orientation selective compared with V1, some showed a bias towards specific orientations (g). (h) Comparison of binocular response and the linear summation of monocular responses in the dLGN. (i) Binocular integration ratio in dLGN. The integration ratio was as high as 3 for very weak responses, but around 1 for all responses larger than 5 spikes per second. Pooled data were presented as mean±s.e.m. Figure 2: Sublinear binocular integration of spiking responses. ( a ) Comparison of binocular spiking response and the linear summation of monocular responses in anaesthetized mice. Most points fell below the unity line, indicating a sublinear binocular integration. ( b ) Comparison of binocular spiking response and the linear summation of monocular responses in awake mice. ( c ) Binocular integration ratio in anaesthetized (black) and awake (blue) conditions. Integration ratio was plotted against the response magnitude, grouped at a bin width of 5 spikes per second. ( d ) A coronal section confirming recording site in the dLGN. The electrode track was marked with DiI (red). Four pictures were assembled to obtain the whole image. The dLGN was approximately marked with a black outline. Scale bar, 400 μm. ( e ) Distribution of ocular dominance index (ODI). Most cells had ODI of 1, indicating that they were monocular. ( f – g ) Two example dLGN cells in response to contralateral (blue), ipsilateral (green) and both eye stimulation (red). One cell was responsive to the contralateral eye ( g ), the other to the ipsilateral eye ( f ). The monocular response did not change much upon opening the other eye for most cells ( f ), but increased for some ( g ). Note that although dLGN cells were much less orientation selective compared with V1, some showed a bias towards specific orientations ( g ). ( h ) Comparison of binocular response and the linear summation of monocular responses in the dLGN. ( i ) Binocular integration ratio in dLGN. The integration ratio was as high as 3 for very weak responses, but around 1 for all responses larger than 5 spikes per second. Pooled data were presented as mean±s.e.m. Full size image V1 is widely accepted as the first stage of binocular convergence. In the dLGN, retinal inputs from the two eyes are anatomically segregated [4] . A few studies in cats and primates, however, reported that binocular interactions exist in the dLGN [23] , [24] , [25] , [26] , probably mediated by local circuits in the dLGN, cortical feedback or connections with other thalamic nuclei (for example, reticular nuclei). We therefore studied binocular responses in the mouse dLGN ( Fig. 2d ). The vast majority of dLGN cells only responded to one eye ( n =14/18; Fig. 2e ), and across population, the binocular responses were similar to the monocular ones ( Fig. 2f ). Interestingly, the response of some cells ( n =7/18) was increased by opening the ‘silent’ eye that did not evoke any response by itself ( Fig. 2g ). This facilitatory effect was more significant for weak responses ( Fig. 2h ). Although the source of this effect remains to be investigated (possible mechanisms include local thalamic circuits and modulatory inputs from the brainstem [27] ), these results clearly demonstrate that the sublinear binocular integration in V1 is derived within the cortex. Sublinear V m integration preserves binocular tuning We next carried out in vivo whole-cell recording of V1 neurons to determine the membrane potential ( V m ) mechanisms underlying the preservation of binocular orientation tuning and the regulation of binocular responsiveness. We classified the recorded neurons into simple and complex by calculating the mean V m depolarization (Δ V 0 ) in response to drifting gratings and the V m ’s first harmonic in Fourier transform (Δ V 1 ) at the drift frequency. Consistent with a report in cats [28] , Δ V 1 /Δ V 0 ratio did not show a bimodal distribution in our recordings. We thus used Δ V 1 /Δ V 0 >0.3 as a cutoff for simple cells ( n =18/62). As shown below, our conclusions are not dependent on this criterion. In addition to the strong and modulated depolarizations at the preferred orientation through each eye (for example, Fig. 3a ), the simple cells also responded at the orthogonal orientation, but the depolarization was smaller and barely modulated (for example, Fig. 3a ). Consequently, the tuning of V m was much broader than that of the spiking ( Fig. 3b ), consistent with previous studies showing that the firing threshold sharpens response selectivity [9] , [10] , [11] . Importantly, the substantial V m depolarizations evoked by the non-preferred orientations raise a problem for preserving binocular orientation tuning. When binocular inputs are summed up, the V m responses at the non-preferred orientations could exceed the threshold and consequently weaken the selectivity of the spiking responses. In other words, the preservation of binocular orientation tuning relies on how V m responses are integrated. 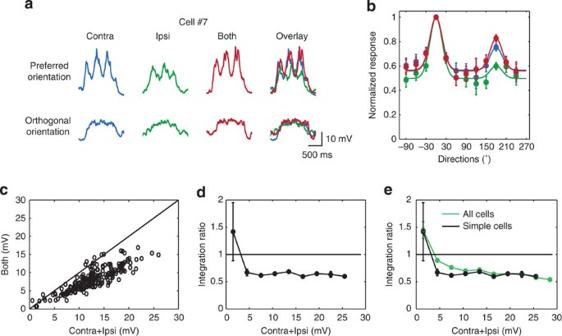Figure 3: Sublinear binocular integration ofVmresponse. (a)Vmtraces of an example cell in response to monocular or binocular stimulation. Substantial depolarizations were evoked at both the preferred and orthogonal directions. In both cases, the binocular responses were only slightly larger than the dominant monocular responses. Spikes were removed from raw traces. (b) Normalized monocular and binocular orientation tuning ofVmresponse (n=18 cells). (c) Relationship between binocularVmresponse and the linear summation of monocular responses, measured by the mean depolarization at each condition. (d) Binocular integration ratio ofVmresponses plotted against the response magnitude (ΔVcontra+ΔVipsi). A bin width of 3 mV was used. (e) Similar integration ratio curves for simple cells (black) and all recorded cells (green). Pooled data were presented as mean±s.e.m. Figure 3: Sublinear binocular integration of V m response. ( a ) V m traces of an example cell in response to monocular or binocular stimulation. Substantial depolarizations were evoked at both the preferred and orthogonal directions. In both cases, the binocular responses were only slightly larger than the dominant monocular responses. Spikes were removed from raw traces. ( b ) Normalized monocular and binocular orientation tuning of V m response ( n =18 cells). ( c ) Relationship between binocular V m response and the linear summation of monocular responses, measured by the mean depolarization at each condition. ( d ) Binocular integration ratio of V m responses plotted against the response magnitude (Δ V contra +Δ V ipsi ). A bin width of 3 mV was used. ( e ) Similar integration ratio curves for simple cells (black) and all recorded cells (green). Pooled data were presented as mean±s.e.m. Full size image We thus examined the mode of binocular integration by plotting the observed binocular V m response against the sum of the two monocular responses at each stimulus orientation. Most data points fell below the unity line ( Fig. 3c ), indicating a sublinear integration. Consistently, the binocular integration ratio for V m response was above 1 only when the depolarization was very weak, and quickly dropped below 1 with increasing response magnitude ( Fig. 3d ). The same mode of binocular integration was seen when all intracellularly recorded cells were included ( Fig. 3e ; n =62), confirming that our criterion of choosing simple cells does not affect the conclusion. We next simulated binocular spiking responses if V m integration were to become linear. The spiking response was simulated by following the cell’s V m -to-spiking transformation function obtained from the experimental data (see Methods and Supplementary Fig. S3 ). As illustrated for an example cell in Fig. 4 , spikes were only observed at seven directions, and the highest at the preferred, 90° ( Fig. 4b ). Although the depolarizations were robust at the other directions, no spiking was evoked. However, if V m integration were linear, spiking responses would be evoked at all conditions ( Fig. 4b ). As a result, the orientation selectivity would become much weaker than the observed, due to the increased baseline ( Fig. 4c ). Consistently, the linear mode of V m integration resulted in significantly smaller OSI and larger CV ( Fig. 4e ). These results reveal that the sublinear V m integration preserves the binocular orientation tuning for spiking, by keeping the depolarization subthreshold at the non-preferred orientations. 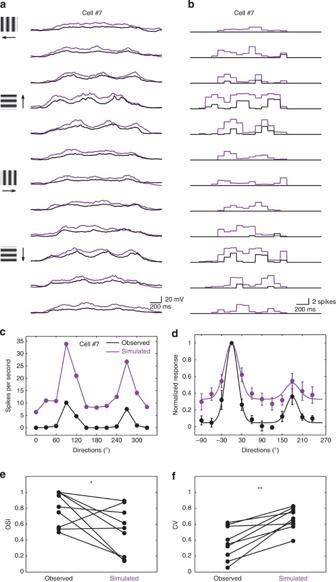Figure 4: SublinearVmintegration preserves binocular orientation tuning. (a) Observed binocularVmresponse (black) and the linear summation of monocular responses (purple) at various directions in an example cell. (b) Observed (black) and simulated (purple) binocular spiking responses in the example cell. The simulated responses were calculated by passing the linear summation of monocularVmresponses through the sigmoidVm-to-spiking transformation function obtained from the experimental data. (c) Orientation tuning curves of the example cell with the observed (black) or simulated (purple)Vmintegration. (d) Mean orientation tuning curves of the observed and simulated responses (n=9 cells). (e) Comparison between the observed and simulated OSIs. OSI was significantly smaller in the linear summation scenario (OSI=0.79±0.07 for the observed and 0.52±0.10 for simulated, mean±s.e.m.,*P<0.05, pairedt-test). (f) Comparison between observed and simulated CVs. CV was significantly larger in the linear summation scenario (CV=0.36±0.07 for the observed and 0.67±0.05 for simulated, **P<0.01, pairedt-test). Pooled data were presented as mean±s.e.m. Figure 4: Sublinear V m integration preserves binocular orientation tuning. ( a ) Observed binocular V m response (black) and the linear summation of monocular responses (purple) at various directions in an example cell. ( b ) Observed (black) and simulated (purple) binocular spiking responses in the example cell. The simulated responses were calculated by passing the linear summation of monocular V m responses through the sigmoid V m -to-spiking transformation function obtained from the experimental data. ( c ) Orientation tuning curves of the example cell with the observed (black) or simulated (purple) V m integration. ( d ) Mean orientation tuning curves of the observed and simulated responses ( n =9 cells). ( e ) Comparison between the observed and simulated OSIs. OSI was significantly smaller in the linear summation scenario (OSI=0.79±0.07 for the observed and 0.52±0.10 for simulated, mean±s.e.m., *P <0.05, paired t -test). ( f ) Comparison between observed and simulated CVs. CV was significantly larger in the linear summation scenario (CV=0.36±0.07 for the observed and 0.67±0.05 for simulated, ** P <0.01, paired t -test). Pooled data were presented as mean±s.e.m. Full size image V m basis of sublinear spiking integration The sublinear V m integration we revealed also provides a basis for the restriction of binocular responsiveness as shown in our extracellular data ( Fig. 2 ). However, other V m mechanisms could also contribute to the sublinear spiking integration. For example, if a simple cell’s responses through the two eyes are out of phase (as seen in disparity tuning in cats and primates [13] ), the binocular spiking response would be significantly lower than the sum of the two monocular responses, even if the V m integration at each time point is linear. In support of this possibility, we found that the recorded simple cells indeed had a small, but non-zero interocular phase difference (median of 31.4°, corresponding to 43.6 ms; n =18; Supplementary Fig. S4a ). Another potential factor in binocular spiking integration is the V m -to-spiking transformation, which was better described by a saturating sigmoid function in our recordings ( Supplementary Fig. S3 ). This was different from the power-law function in cats [28] , in which the slope monotonically increases. The ‘ceiling effect’ in the sigmoid V m -to-spiking transformation could in theory contribute to the sublinear binocular integration of spiking responses. We sought to reveal the relative contributions of sublinear V m integration, sigmoid V m -to-spiking transformation and interocular phase difference to binocular integration of spiking responses. We focused our analysis on the preferred orientation, at which the last two factors were potentially prominent. We again simulated spiking responses just as in the previous section, and altered each of the three factors independently while keeping the others unchanged. For example, if the V m integration were linear, the binocular spiking response would dramatically increase ( Fig. 5e–i ), just as shown in Fig. 4 . In fact, all neurons would have an integration ratio larger than 1 ( n =6/6 compared with n =2/6 as observed), resulting from the supralinear V m -to-spiking transformation. In contrast, removing the interocular phase difference by temporally aligning the peaks of the monocular responses, and changing the V m -to-spiking function from sigmoid to power law did not cause a significant increase of the integration ratio ( Fig. 5j–s ). This analysis thus demonstrates that the sublinear binocular integration of spiking response is primarily due to the sublinear V m integration. 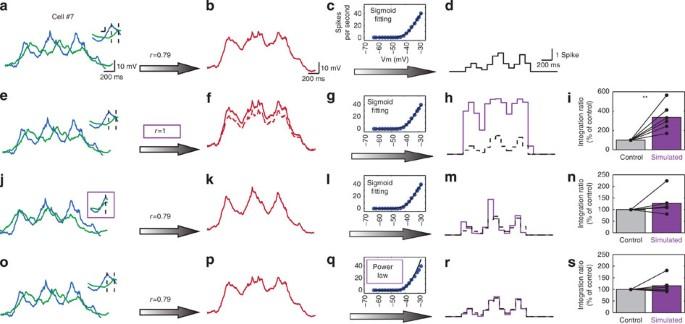Figure 5: Sublinear binocular integration of spiking is primarily due to sublinearVmintegration. (a–d) Control condition. The recorded monocularVmresponse traces at the preferred orientation (a) were added and multiplied with theVmintegration ratio determined from the experimental data to predict binocularVmresponse (b). The interocular phase shift was shown by a cycle average of theVmresponses (a, inset figure scale bars, 5 mV and 100 ms). The simulated binocularVmresponse was then binned at 100 ms and passed through the sigmoidVm-to-spiking transformation function (c) to calculate spiking rate at each bin (d). (e–h) LinearVmintegration. The same procedure was followed as ina–d, except that a binocular integration ratio of 1 was used (marked by the purple box).Vmand spiking responses of the control model was reproduced by the dotted lines infandhfor comparison. (i) LinearVmintegration would increase binocular integration ratio of spiking response by 235% (P<0.01, pairedt-test,n=6). (j–m) Aligned interocular phase. The same procedure as ina–d, except that the monocular responses were temporally shifted to align their peaks (marked by the purple box). (n) Aligning interocular phase only increased the integration ratio by 27% (P=0.27, pairedt-test,n=6). (o–r) Power-law transformation. The same procedure as ina–d, except that theVm-to-spiking transformation was changed to a power-law function fitted by the initial part of data points (marked by the purple box). (s) A power-law transformation only increased integration ratio by 16% (P=0.25, pairedt-test,n=6). Figure 5: Sublinear binocular integration of spiking is primarily due to sublinear V m integration. ( a – d ) Control condition. The recorded monocular V m response traces at the preferred orientation ( a ) were added and multiplied with the V m integration ratio determined from the experimental data to predict binocular V m response ( b ). The interocular phase shift was shown by a cycle average of the V m responses ( a , inset figure scale bars, 5 mV and 100 ms). The simulated binocular V m response was then binned at 100 ms and passed through the sigmoid V m -to-spiking transformation function ( c ) to calculate spiking rate at each bin ( d ). ( e – h ) Linear V m integration. The same procedure was followed as in a – d , except that a binocular integration ratio of 1 was used (marked by the purple box). V m and spiking responses of the control model was reproduced by the dotted lines in f and h for comparison. ( i ) Linear V m integration would increase binocular integration ratio of spiking response by 235% ( P <0.01, paired t -test, n =6). ( j – m ) Aligned interocular phase. The same procedure as in a – d , except that the monocular responses were temporally shifted to align their peaks (marked by the purple box). ( n ) Aligning interocular phase only increased the integration ratio by 27% ( P =0.27, paired t -test, n =6). ( o – r ) Power-law transformation. The same procedure as in a – d , except that the V m -to-spiking transformation was changed to a power-law function fitted by the initial part of data points (marked by the purple box). ( s ) A power-law transformation only increased integration ratio by 16% ( P =0.25, paired t -test, n =6). Full size image Synaptic inhibition promotes sublinear binocular integration We next studied what cellular mechanisms give rise to the sublinear binocular integration of V m . First, the observed sublinear V m integration was not due to action potential shunting ( Supplementary Fig. S5 ). Another biophysical property that could contribute to the nonlinear V m integration is the driving force. With V m getting closer to the reversal potential of the synaptic input, the driving force is reduced. As a result, additional increase in synaptic conductance ( g ) would evoke less current and V m change. Importantly, the closer the reversal potential is to V m , the more significant g -to- V m nonlinearity will be. Because neurons receive both excitatory and inhibitory inputs in response to visual stimulation, the effective reversal potential ( E syn ) is determined by the excitatory and inhibitory reversal potentials ( E ex and E inh ) weighted by their conductances ( g ex and g inh ): Because E inh is very close to the resting V m , synaptic inhibition should have a large impact on V m integration, where larger inhibition (that is, g inh ) would lead to a more hyperpolarized E syn , and consequently more sublinear V m integration. Importantly, to profoundly affect V m integration, g inh needs to overlap with g ex temporally. To determine if this was indeed the case, we recorded visually evoked inhibitory post-synaptic potentials (IPSPs) and excitatory post-synaptic potentials (EPSPs) at each cell’s preferred orientation ( Supplementary Fig. S6c ), under current clamp with Cs + -based internal solution. The visually evoked changes in synaptic conductances were then estimated based on a passive neuron model (see Methods for details). The excitatory and inhibitory conductances in simple cells displayed phasic temporal dynamics following the drifting gratings ( Fig. 6a ). The time courses of g ex and g inh were similar between the two eyes (that is, in-phase) ( Fig. 6a , |ΔPhase|=28.7±7.7° for excitation and 36.3°±8.1° for inhibition, mean±s.e.m. ), consistent with the V m data. Importantly, in the majority of recorded cells, binocularly evoked g ex and g inh were largely in-phase, consistent with previous studies of contralaterally evoked responses in mice [10] , [11] ( n =6/9 cells having |ΔPhase|<90°, mean of 60.4±17.5°). We then calculated binocularly evoked total synaptic conductance changes ( Δg = Δg ex + Δg inh ) for each cell. As expected from the largely in-phase excitation and inhibition, Δg showed strong modulation within each stimulus cycle ( Fig. 6b ), with its peak (11.0±1.9 nS, n =9) larger than the mean input conductance (9.8±2.7 nS, n =15), which was measured from a separate set of current-clamp experiments with K + -based internal solution. In other words, overlapping excitation and inhibition double the cell's membrane conductance at the peak of binocular response, which would induce a large reduction in the driving force. 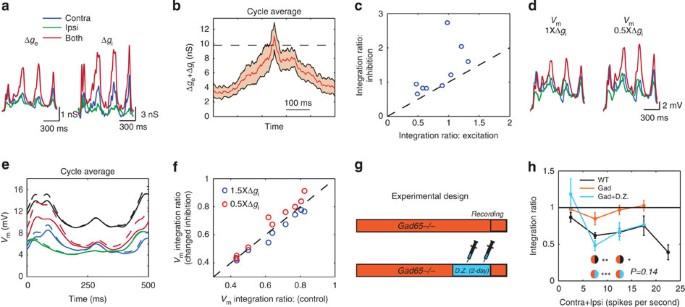Figure 6: Inhibition promotes sublinear binocular integration. (a) Changes in excitatory (Δge) and inhibitory conductances (Δgi) at the preferred orientation in an example cell. (b) Cycle average of total conductance change (Δg=Δgi+Δgi) in response to binocular stimulation. The mean (red line) and the s.e.m. (light red area) of Δgwas plotted (n=9). The mean input conductance of simple cells (n=15), measured from a separate set of experiments, was marked by the dashed black line. (c) Binocular integration ratio of excitatory and inhibitory conductances. Black dashed lines marked the unity line. Note that inhibition showed significantly higher integration ratios than excitation (P<0.05, pairedt-test). (d) An example of simulated monocular and binocularVmresponses using the experimentally estimated conductances (left), or using 50% of inhibition (0.5 × Δgi, right). (e) The same example as ind, showing the cycle average ofVmdepolarizations. Results of the control condition were plotted in solid lines, and 0.5 × Δgicondition in dashed lines. Blue, green and red colours represent contralateral, ipsilateral and both eyes, respectively, just as in other panels and figures. The linear sums of monocular responses were plotted with black lines. Note that the change of binocular response (red solid versus red dashed) was greater than that of monocular responses (black solid versus black dashed). (f) Population data of simulatedVmintegration ratios with increased (blue) or decreased (red) inhibition plotted against the control condition (P<0.05 for 1.5 × Δgiversus control andP<0.01 for 0.5 × Δgiversus control). The black dashed line marked the unity line.Vmresponses were quantified as the peaks of cycle averaged simulatedVmresponses. (g–h) Binocular integration ratio inGad65−/− and diazepam-treated mice. Two doses of diazepam (D.Z.) were injected at 24 h apart and the mice were then recorded 24 h later (g). Integration ratio curves of spiking response for wild-type,Gad65−/−andGad65−/−with D.Z. injection are shown inh. In the second bin, ***P<0.001 forGadversus WT and **P<0.01 forGadversusGad+DZ; in the third bin, *P<0.05 forGadversus WT andP=0.14 forGadversusGad+DZ, Mann–Whitney test; too few data points are in the fourth bin to allow statistical test. Pooled data were presented as mean±s.e.m. Figure 6: Inhibition promotes sublinear binocular integration. ( a ) Changes in excitatory (Δ g e ) and inhibitory conductances (Δ g i ) at the preferred orientation in an example cell. ( b ) Cycle average of total conductance change (Δ g =Δ g i +Δ g i ) in response to binocular stimulation. The mean (red line) and the s.e.m. (light red area) of Δ g was plotted ( n =9). The mean input conductance of simple cells ( n =15), measured from a separate set of experiments, was marked by the dashed black line. ( c ) Binocular integration ratio of excitatory and inhibitory conductances. Black dashed lines marked the unity line. Note that inhibition showed significantly higher integration ratios than excitation ( P <0.05, paired t -test). ( d ) An example of simulated monocular and binocular V m responses using the experimentally estimated conductances (left), or using 50% of inhibition (0.5 × Δ g i , right). ( e ) The same example as in d , showing the cycle average of V m depolarizations. Results of the control condition were plotted in solid lines, and 0.5 × Δ g i condition in dashed lines. Blue, green and red colours represent contralateral, ipsilateral and both eyes, respectively, just as in other panels and figures. The linear sums of monocular responses were plotted with black lines. Note that the change of binocular response (red solid versus red dashed) was greater than that of monocular responses (black solid versus black dashed). ( f ) Population data of simulated V m integration ratios with increased (blue) or decreased (red) inhibition plotted against the control condition ( P <0.05 for 1.5 × Δ g i versus control and P <0.01 for 0.5 × Δ g i versus control). The black dashed line marked the unity line. V m responses were quantified as the peaks of cycle averaged simulated V m responses. ( g – h ) Binocular integration ratio in Gad65 −/− and diazepam-treated mice. Two doses of diazepam (D.Z.) were injected at 24 h apart and the mice were then recorded 24 h later ( g ). Integration ratio curves of spiking response for wild-type, Gad65−/− and Gad65−/− with D.Z. injection are shown in h . In the second bin, *** P <0.001 for Gad versus WT and ** P <0.01 for Gad versus Gad +DZ; in the third bin, * P <0.05 for Gad versus WT and P =0.14 for Gad versus Gad +DZ, Mann–Whitney test; too few data points are in the fourth bin to allow statistical test. Pooled data were presented as mean±s.e.m. Full size image We also quantified binocular integration ratio for excitatory and inhibitory conductances. The integration ratio of g ex was smaller than 1 in some cells ( Fig. 6c ), presumably caused by intracortical inputs that were already sublinear in their binocular integration. Interestingly, the integration ratio of g inh was higher than that of g ex in almost every cell ( Fig. 6c ), which would lead to a lower E / I ratio and consequently smaller V m depolarization in response to binocular stimulation. To explore what might cause the difference in integration ratio between g ex and g inh , we identified putative fast-spiking interneurons from extracellular recordings based on their spike waveforms ( Supplementary Fig. S7 ). The integration ratio of the putative fast-spiking interneurons was indeed significantly higher than that of excitatory cells, especially the simple cells ( Supplementary Fig. S7d ). Although the origin of this cell-type-specific integration remains to be investigated, our analysis reveals another way for cortical inhibition to contribute to sublinear binocular integration. To illustrate the effect of synaptic inhibition on binocular integration, we simulated V m responses using the measured synaptic conductances for each cell, and altered the strength of Δg inh . With the experimentally observed integration ratio, the simulated change of inhibition was thus in proportion across monocular and binocular conditions. As expected, decreasing inhibition by 50% slightly increased the monocular V m responses ( Fig. 6d ). Importantly, consistent with the driving force nonlinearity, the increase of binocular response was even greater. This was reflected by the significantly increased integration ratio across the population, and the opposite effect was seen when inhibition was increased by 50% ( Fig. 6f ). Although the change of V m integration was small in our simulation, it could result in a profound change in spiking due to the threshold and superlinear V m -to-spiking transformation function (c.f. Fig. 5f ). To experimentally test this possibility, we recorded simple cells in mutant mice that lack 65 kDa glutamic acid decarboxylase (Gad65), an essential enzyme for GABA synthesis [29] . These mice have lower GABA concentration and thus compromised inhibition level [30] , [31] , which was shown previously to sufficiently affect their visual responses [31] , [32] . Gad65 −/− mice indeed showed significantly higher integration ratios ( Fig. 6h ). To rule out possible complicating effects of the mutation such as developmental compensation, we tested whether the altered integration ratio in the Gad65 −/− mice could be restored by increasing the level of inhibition. Administration of the use-dependent GABA-A receptor agonist diazepam can chronically increase the inhibition level in the Gad65 −/− mice [30] , [31] , [32] , [33] , [34] , probably by triggering GABA-A receptor insertion at peri-somatic sites [33] . We treated adult Gad65 −/− mice with intraperitoneal injections of diazepam (30 mg g −1 ) twice at a 24-h interval, and then recorded one day later after the second injection ( Fig. 6g ). Remarkably, diazepam treatment reduced the mutant’s integration ratio to the level of wild-type mice ( Fig. 6h ). Together, these results demonstrate that inhibition indeed has a critical role in the sublinear integration of binocular responses. We next examined the effect of reducing inhibition on binocular orientation tuning. The binocular tuning curve in the Gad65 −/− mice was closer to the summed monocular curves and above the binocular tuning curve in wild type ( Supplementary Fig. S8a,b ), consistent with the increased integration ratio. However, there was only a slightly elevated baseline in the Gad65 −/− ( Supplementary Fig. S8c ). The lack of a large change in binocular orientation tuning was likely due to the extent of inhibition reduction in these mutants. With increased V m integration ratio, the depolarization at non-preferred orientations, even though now larger, may still be subthreshold. On the other hand, a small increase in the above-threshold V m responses at the preferred orientations would lead to a large increase in firing rates due to the supralinear V m -to-spiking transformation. To conceptually illustrate this point, we constructed a simple receptive-field based model ( Supplementary Fig. S9a and see Supplementary Methods for details) with different excitation/inhibition ratios [35] . Twenty per cent reduction in inhibition led to a dramatic increase in the integration ratio but only changed the binocular tuning curve slightly ( Supplementary Fig. S9b,c ). Reducing inhibition by another 20%, in contrast, caused a much more broadening in tuning ( Supplementary Fig. S9d ). It is therefore likely that the recorded Gad65−/− mutants only bore a moderate reduction in inhibition, which affected binocular integration without significantly broadening the tuning. Contribution of callosal projections to binocular integration In addition to the feed-forward thalamocortical pathway, visual stimulation may also activate interneurons through other pathways, such as inter-hemispherical projections. The two cortical hemispheres are connected via excitatory transcallosal axons. The functional effect of the callosal projections, however, could be inhibitory through multi-synaptic connections, as demonstrated in the somatosensory cortex [36] , motor cortex [37] and frontal lobe [38] . We thus examined the potential contribution of callosal projections to binocular integration. In each animal, a single unit was recorded before and after silencing V1 of the other hemisphere with tetrodotoxin (TTX) ( Fig. 7a ). The removal of callosal input increased the contralateral eye’s response in some cells (for example, Fig. 7b ) and decreased in others, without a significant trend ( Fig. 7d , P >0.5, n =9 cells). In contrast, the ipsilateral eye’s response was consistently and significantly reduced by removing the callosal input, indicating that the net effect of the callosal input is excitatory ( Fig. 7c , P <0.01). This finding is consistent with a previous report that callosal projections contribute to visually evoked local field potentials (VEPs) through the ipsilateral, but not the contralateral eye [39] , also confirming that the TTX effect in our experiment was limited to the treated hemisphere. More importantly to our current study, the binocular integration ratio did not change after removal of the callosal input ( Fig. 7f , P >0.5). In other words, unlike in the somatosensory cortex where the two hemispheres suppress each other [36] , the inter-hemispherical interaction between V1 affects ocular dominance by enhancing ipsilateral eye response, without changing the sublinear binocular integration. 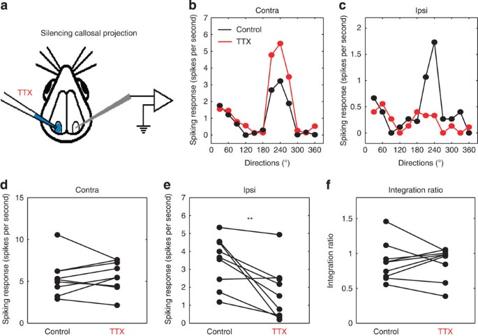Figure 7: Callosal projections contribute to ipsilateral eye responses but do not affect binocular integration. (a) Experimental design. Monocular and binocular responses of single units were studied before and after 0.3–0.5 μl TTX (200 nM) was injected to silence V1 on the other side. (b,c) Monocular spiking responses of an example cell before (black) and after (red) TTX injection. (d,e) Comparison of monocular response magnitude at the preferred orientation before and after TTX injection. The response through the contralateral eye was not significantly affected (5.0±0.8 spikes per second before and 5.1±0.8 spikes per second after,P>0.5, pairedt-test), while the ipsilateral response was reduced after silencing the other hemisphere (3.3±0.5 spikes per second before and 1.5±0.5 spikes per second after,n=9, **P<0.01, pairedt-test). (f) Comparison of binocular integration ratios before and after TTX injection. No significant difference was seen (0.88±0.09 before and 0.79±0.11 after,P>0.5, pairedt-test). Figure 7: Callosal projections contribute to ipsilateral eye responses but do not affect binocular integration. ( a ) Experimental design. Monocular and binocular responses of single units were studied before and after 0.3–0.5 μl TTX (200 nM) was injected to silence V1 on the other side. ( b , c ) Monocular spiking responses of an example cell before (black) and after (red) TTX injection. ( d , e ) Comparison of monocular response magnitude at the preferred orientation before and after TTX injection. The response through the contralateral eye was not significantly affected (5.0±0.8 spikes per second before and 5.1±0.8 spikes per second after, P >0.5, paired t- test), while the ipsilateral response was reduced after silencing the other hemisphere (3.3±0.5 spikes per second before and 1.5±0.5 spikes per second after, n =9, ** P <0.01, paired t- test). ( f ) Comparison of binocular integration ratios before and after TTX injection. No significant difference was seen (0.88±0.09 before and 0.79±0.11 after, P >0.5, paired t- test). Full size image Binocular cortical cells usually receive inputs simultaneously through both eyes, but the circumstance under which only one eye is activated can also occur naturally. An object may block one eye’s view, while leaving the other eye unaffected. In humans, binocular vision performs equally well as monocular vision in an orientation discrimination task with strong stimuli [40] . The sublinear V m integration that we discovered here gives simple cells the ability to have similar orientation tuning for both monocular and binocular vision, providing a physiological basis for the psychophysical observations. The sublinear V m integration also led to a restriction of binocular responsiveness, which may prevent V1 and downstream visual centres from saturation. The cellular mechanism revealed in this study may also apply to other sensory processes, in which the system can switch effortlessly between single and multiple input channels. In cats, the majority of simple cells showed linear or supralinear binocular integration of spiking responses at the preferred orientation [1] , [41] . This difference may result from the different dynamics of excitatory and inhibitory responses to drifting gratings between the two species. At the preferred orientations, the excitatory and inhibitory inputs to simple cells are out-of-phase in cats, but in-phase in mice [11] . As a result, in cats, the input is mostly free of inhibition at the depolarization peak, allowing higher integration ratio when more inputs are added. It should be noted that this temporal shift between excitation and inhibition is only prominent at the preferred orientations. At other orientations, excitation and inhibition are mainly comprised of a DC component and correlate temporally in both species. Therefore, sublinear V m integration may also have a role in preserving binocular orientation tuning in higher mammals by suppressing spiking at non-preferred orientations. Mouse eyes are located more laterally than in carnivores and primates, but there is still a significant binocular visual field (~30° on each side of vertical meridian) [42] . A behavioural study suggested that mice may use binocular vision to estimate the distance to an object [43] . At the physiological level in mice, the two monocular receptive fields of individual simple cells overlap spatially and have similar subregion layout [44] . Consistently, mouse V1 cells are tuned to similar orientations through the two eyes [8] , just like in higher mammals [6] , [7] . Importantly, the binocular matching of orientation preference in mice requires binocular visual experience during postnatal development [8] , suggesting that correlated images are indeed seen by the two eyes in this species. The sublinear V m integration could also improve disparity tuning ( Supplementary Fig. S10 ), an important function for stereo vision. It is important to note that the V m modulation in mice was relatively small in most cells even at the preferred orientation (for example, Fig. 3a ). The small modulation is expected from the lack of a push–pull organization of excitation and inhibition seen in cats [10] , [11] , and renders V m summation less sensitive to phase disparity. This observation can thus account for the broader disparity tuning in mice [45] . The preservation of binocular orientation tuning is computationally analogous to contrast invariance, a well-studied phenomenon in V1. Both processes face the same problem: to prevent the cell from losing its response selectivity when input strength increases [46] . Inhibition-based models have been proposed to explain contrast invariance [47] , [48] . Intracellular data in cats, however, support a feed-forward mechanism with contrast-modulated V m variability that originates from dLGN relay cells [49] . In contrast, the preservation of binocular orientation tuning is implemented in a different way. Binocular response properties rely largely on cortical computation, as inputs from the two eyes first converge in V1. For example, interocular cross-orientation suppression was shown to recruit intracortical inhibition [16] , while monocular cross-orientation suppression can arise from the feed-forward inputs from the dLGN [50] . Indeed, we showed that the sublinear binocular integration is not seen in the dLGN, but instead takes place in the cortex and is enhanced by cortical inhibition. The role of cortical inhibition in generating monocular visual responses has been extensively studied in cat V1 over the past several decades, and more recently in mice. The combined feed-forward excitatory input to simple cells is already orientation selective [10] , [11] , [51] , [52] , and cortical inhibition determines the cell’s spiking response by regulating its input–output transformation function [10] , [18] , [20] , [53] . Our result is consistent with this general principle, and extends it to binocular vision. With simple cells tuned to similar orientations through the two eyes, the converging inputs under binocular stimulation are biased towards the preferred orientation. Inhibition controls binocular integration ratio through the driving force effect and in turn determines the spiking output. Animal preparations Young adult (P35-P50) and adult (P60-P90) wild-type C57BL/6 mice, both genders, were used in the experiments. No significant difference was seen between the two age groups and they were pooled together in data analysis. Gad65 knockout mice were obtained from Jackson Laboratory (Stock no. 003654). The colony was maintained by crossing heterozygotes ( Gad65+/− ) with wild-type mice. Heterozygotes were bred and genotyped to produce homozygous offspring for recording. All experimental procedures were approved by Northwestern University Institutional Animal Care and Use Committee. In anaesthetized recordings, mice were sedated with chlorprothixene (5 mg kg −1 in water, intraperitoneally (i.p.)) and then anaesthetized with urethane (1–1.25 g kg −1 in 10% saline solution, i.p.). Atropine (0.3 mg kg −1 , in 10% saline) and dexamethasone (2 mg kg −1 , in 10% saline) were administrated subcutaneously, as described before [8] , [44] , [54] , [55] . Throughout recordings, toe-pinch reflex was monitored and additional urethane (0.2–0.3 g kg −1 ) was supplemented as needed. In extracellular recordings, the animal was seated in a stereotaxic apparatus. In whole-cell recordings, a metal head plate was implanted on top of the skull with dental cement, and the plate was then mounted to a stand on the recording table. In both cases, the animal’s temperature was monitored with a rectal thermoprobe and maintained at 37 °C through a feedback heater control module (Frederick Haer Company, Bowdoinham, ME). Silicon oil was applied on both eyes to prevent from drying. In cortical recordings, a small craniotomy (~2 mm 2 ) was drilled on the left hemisphere to expose V1. The centre of the craniotomy was 3 mm lateral and 0.5 mm anterior from the lambda point. In the experiments to manipulate callosal projections, a second craniotomy was done on the other hemisphere for drug injection. In dLGN recordings, the craniotomy was 2 mm lateral and 2.6 mm posterior from the Bregma point. In awake recordings, mice were first anaesthetized with isoflurane (~1%) to implant a head plate with MetaBond (Parkell, Inc). Carprofen (1 g kg −1 in 10% saline solution) was injected subcutaneously after the surgery. On the second day, the animal was anaesthetized again with isoflurane and craniotomy performed. The exposed cortex was protected with Kwik-Sil adhesive (World Precision Instruments). The animal was then let to recover from the anaesthesia for at least 1 h, and was placed in a holder via the head plate. The animal’s body was restricted in a plastic tube. In vivo extracellular recording Tungsten electrodes (5–10 MΩ, FHC) were inserted perpendicular to the pial surface. Cortical cells were recorded between 150 μm and 500 μm in depth, corresponding to layer 2/3 and layer 4. LGN cells were recorded between 2.4 mm and 3.0 mm below the surface. In experiments where the depth of layer 4 was determined, we mapped current source density (CSD) by recording VEPs at 14 different depths (0–650 μm, at 50 μm spacing), after finishing single-unit recordings of each individual penetration. CSD was calculated as the second-order spatial derivative of VEPs, as described before [17] . Layer 4 was identified by a fast and strong current sink, indicating its strong feed-forward input. The identified layer 4 ranged between 250 μm and 450 μm in most penetrations. Electrical signals were filtered between 0.3 and 5 kHz for spikes, and 10 and 300 Hz for VEPs and sampled at 25 kHz using a System 3 workstation (Tucker Davis Technologies, FL). The spike waveforms were sorted offline in OpenSorter (Tucker Davis Technologies, FL) to isolate single units. In vivo whole-cell recording Blind patch clamp was performed to record cortical cells intracellularly as described previously [10] , [28] . Glass pipettes had tip openings of 1.5–2 μm (6–10 MΩ). For recording V m dynamics, the internal solution contained 135 mM K-gluconate, 4 mM KCl, 0.5 mM EGTA, 10 mM HEPES, 10 mM Na-phosphocreatine, 4 mM Mg-ATP and 0.4 mM GTP. The pH was adjusted to 7.2 with KOH. For estimating synaptic conductances, the internal solution contained 125 mM Cs-gluconate, 2 mM CsCl, 0.5 mM EGTA, 10 mM HEPES, 1 mM QX-314, 5 mM TEA-Cl, 10 mM Na-phosphocreatine, 4 mM Mg-ATP and 0.4 mM GTP. The pH was adjusted to 7.2 with gluconic acid. Cs + , TEA and QX-314 were to minimize currents from voltage-gated K + and Na + channels to isolate synaptic events. After inserting the pipette into the cortex, 2.5% agarose in artificial cerebrospinal fluid was applied on top of the cortex to reduce pulsation. Signals were amplified using MultiClamp 700B (Axon Instruments, CA), sampled at 10 kHz. The signal was then acquired with System 3 workstation (Tucker Davis Technologies, FL). Pipette capacitance and the open tip resistance were compensated initially. After the whole-cell configuration was achieved, the membrane potential was recorded under current-clamp mode. To analyse V m integration, no holding current was used unless specified. To estimate synaptic conductances, V m was recorded under two different holding currents, which maintained the cell’s at ~−70 mV and +20 mV to reveal EPSP and IPSP, respectively. A 150-ms square pulse of 55 pA hyperpolarizing current was injected within each stimulus interval to measure membrane and pipette properties (see Data Analysis below for details). Only cells with stable resting membrane potentials were included in our analysis. Visual stimuli Sinusoidal gratings drifting perpendicular to their orientations were generated with Matlab Psychophysics toolbox [56] , [57] , as described previously [8] , [17] . Stimuli were presented using a cathode ray tube monitor (40 × 30 cm, 60 Hz refresh rate, ~35 cd m −2 luminance) 25 cm in front the animal. The orientation of gratings varied between 0° and 330° (12 steps at 30° spacing) in a pseudorandom sequence. In extracellular recordings, the spatial frequency varied between 0.01 and 0.08 cycle per degree (four logarithmic steps). In whole-cell recording, spatial frequencies of 0.02 and 0.04 cycle per degree were used. Temporal frequency was fixed at 2 cycle per second. Each stimulus was presented for 1.5 s (3 cycles), with 0.5 s inter-stimulus interval. Data analysis To identify simple cells in extracellular recordings, we calculated the ratio between the response’s first harmonic at the stimulus drift frequency ( F 1 ) and the mean response ( F 0 ). In anaesthetized animals, we used a standard criterion, F 1 / F 0 >1 for each eye, to classify simple cells. In awake animals, the response timing was more variable from trial to trial. As a result, F 1 / F 0 tended to be smaller than in the anaesthetized condition. We thus used a looser criteria, F 1 / F 0 >0.8, which identified 40% ( n =12/30) of our total recordings as simple cells, similar to the percentage of simple cells in the anaesthetized condition (45%, n =27/60). In intracellular recordings, the modulation ratio was calculated using the V m response (Δ V 1 /Δ V 0 ). We used Δ V 1 /Δ V 0 >0.3 as the cutoff to classify simple cells. To calculate the spiking response ( R spike ), spontaneous spiking rate was subtracted from the total rate at each stimulus condition. For analysing subthreshold responses in intracellular recordings, spikes were first removed from the recorded voltages traces (see Supplementary Methods for details). The V m response ( R v ) was calculated by subtracting the mean V m during a 200-ms window before the stimulus from the mean V m during the stimulation. Binocular integration ratio was calculated as the ratio of R both /( R contra + R ipsi ). Only data points with positive response magnitudes ( R contra + R ipsi >0) were included in the analysis. Preferred orientation (pref_θ) was defined as the stimulus orientation that evoked the maximal response. To be consistent, we defined the pref_θ of a cell using its binocular tuning curve. As shown previously [8] and in this study ( Supplementary Fig. S1 ), most cells had matched pref_θ through the two eyes. Therefore, the binocular pref_θ also matched with the monocular ones in most cells. In the analyses that required more accurate estimation of the preferred orientation, pref_ θ fit was obtained by calculating the half of the complex phase of Σ R(θ)e 2iθ /ΣR(θ) , which is the mean of stimulus orientations weighted by response magnitudes. To obtain the normalized tuning curve, response (spiking rates for extracellular recordings and mean depolarizations for intracellular recordings) across all directions were normalized by the one at the preferred direction, and each cell’s preferred direction was shifted to be aligned. OSI and CV were calculated to quantify orientation tuning (see Supplementary Methods for details). V m -to-spiking transformation was fitted with sigmoid function: where r is the spiking rate, r max the maximal spiking rate, v the membrane potential, v th the threshold, d 1/2 the half peak depolarization and k the slope coefficient. To estimate the synaptic conductance change from the recorded EPSPs and IPSPs, we adopted the passive single compartment model widely used in previous studies [11] , [58] : where V r is the resting membrane potential, Δ g ex the change of excitatory conductance, Δ g inh the change of inhibitory conductance, E ex the equilibrium potential for excitation and E inh the equilibrium potential for inhibition. We assumed E ex =0 mV and E inh =−80 mV, and V , V r , C m and R in were measured from the experiment (see Supplementary Methods for details). The voltage offset caused by the series resistance was corrected: With two holding currents (two sets of V and V r ), Δg ex and Δg inh were solved from the equations. To simulate V m with the conductance data, we used the same equation of passive single compartment model described above. Δg ex and Δg inh were taken from our experimental data and smoothed with a Gaussian filter (s.d. of 10 ms). Other parameters were: V r =−80 mV, C m =83 pF, R in =120 MΩ, E ex =0 mV and E inh =−80 mV. How to cite this article: Zhao, X. et al. Sublinear binocular integration preserves orientation selectivity in mouse visual cortex. Nat. Commun. 4:2088 doi: 10.1038/ncomms3088 (2013).